Identification of vertebra-like elements and their possible differentiation from sclerotomes in the hagfish The hagfish, a group of extant jawless fish, are known to lack true vertebrae and, for this reason, have often been excluded from the group Vertebrata. However, it has yet to be conclusively shown whether hagfish lack all vertebra-like structures, and whether their somites follow developmental processes and patterning distinct from those in lampreys and gnathostomes. Here we report the presence of vertebra-like cartilages in the in-shore hagfish, Eptatretus burgeri . These elements arise as small nodules occupying anatomical positions comparable to those of gnathostome vertebrae. Examination of hagfish embryos suggests that the ventromedial portion of a somite transforms into mesenchymal cells that express cognates of Pax1/9 and Twist , strikingly similar to the pattern of sclerotome development in gnathostomes. We conclude that the vertebra-like elements in the hagfish are homologous to gnathostome vertebrae, implying that this animal underwent secondary reduction of vertebrae in most of the trunk. Vertebrae arise as segmental endoskeletal elements associated with the notochord, and are regarded as a vertebrate synapomorphy [1] , [2] , [3] , [4] , [5] . No such structures, nor the somite-derived vertebral primordial, the sclerotome, are present in non-vertebrate chordates such as amphioxus and the tunicates [6] , [7] . The vertebrae in gnathostomes, the jawed vertebrates, consist of dorsal and ventral elements [1] , [2] , [3] , [4] , [5] , [8] , [9] , [10] , of which only the dorsal elements are present in lampreys [11] , one of the two extant agnathan taxa (jawless fishes) [1] , [2] . Based on evidence that the vertebrae of the gnathostomes and lampreys are developmentally derived from the sclerotome [12] , [13] , it is thought that their developmental mechanisms share the same ancestral origin. However, another extant agnathan, the hagfish, has generally been thought to lack vertebrae; the axial supporting tissue of this animal has been described as consisting only of notochord and cartilaginous fin rays [1] , [2] , [3] , [4] , [14] , [15] , [16] , [17] . Because of this morphological trait, the hagfish was excluded from the Vertebrata in some textbooks [1] , [2] , [5] , although its vertebrate affinities, as observed in the brain and skull, are widely recognized [1] , [2] , [3] , [4] , [5] . This raises a number of questions; specifically, whether the hagfish truly lacks any form of vertebra-like structure throughout its body and life cycle, and whether hagfish somites in the embryonic trunk are dissimilar to those in lampreys and gnathostomes. Importantly, one of the early reports on hagfish anatomy, in fact, described segmental cartilaginous elements (putative vertebral elements) on the ventral aspect of the caudal notochord in Bdellostoma more than a century ago ( Supplementary Fig. S1 ) [18] . These cartilaginous structures have not been re-examined, and have largely been overlooked by subsequent researchers [16] , [17] . To address these questions, we conducted detailed anatomical and histological analyses on the in-shore Japanese hagfish, Eptatretus burgeri , and discovered putative vertebral elements in the caudalmost region of the body axis. These skeletal elements are small cartilaginous nodules mostly located on the ventral aspect of the notochord, reminiscent of the gnathostome hemal arch, which, if not segmented, are in register with myomeres. Furthermore, we obtained a series of early- to late-stage hagfish embryos. Their examination suggests that the ventromedial portions of somites transform into mesenchymal cell masses that express cognates of Pax1/9 and Twist , similar to vertebral primodia in gnathostomes [12] . On the basis of these observations, we propose that the apparent lack of vertebrae in the hagfish stems from secondary developmental suppression of the vertebral differentiation programme for most of the trunk somites. The adult skeletal morphology In adult specimens of E. burgeri , we found putative vertebral elements in the post-cloacal axis ( Fig. 1a–e ) [18] . Histochemical observation indicated that these structures were cartilaginous nodules; the chondrocytes in each nodule were separated by a thin layer of extracellular matrices that were stained with Alcian blue, which detects mucopolysaccharides, as in gnathostomes ( Figs 1c–e and 2a,b ) [2] , [19] . These cartilages consisted of a pair of elements on both sides of the dorsal aorta, a single median element beneath the aorta, and another pair adhering to the ventral aspect of the notochordal sheath ( Fig. 1c,d ). The distribution of these nodules was restricted to a part of the post-cloacal region that roughly corresponded to the position between the 80th and 100th myomeres and was dorsal to the mucus glands ( Fig. 1a,b ). Unlike the vertebrae of lampreys and gnathostomes ( Fig. 2c–f ), these cartilages did not show a clear segmental pattern in register with myomeres. The overall morphology of these elements was reminiscent of hemal arches in gnathostomes ( Figs 1c and 2a,e ) [1] , [2] . On the dorsal side of the notochord at the same axial level, the median plate-like cartilaginous element was associated with dorsal fin rays, which were also present at the post-cloacal level of the trunk. This cartilage was previously designated as the 'median dorsal bar' [18] . As seen in the transverse section of the most caudal level, the median dorsal bar was attached to a pair of cartilaginous arches on both sides of the notochord ( Fig. 1e ). The anatomical configuration of these cartilages is strikingly reminiscent of the neural spine and the paired neural arches in gnathostomes ( Fig. 2e ) [1] , [2] , [3] , [4] , [5] , [18] . 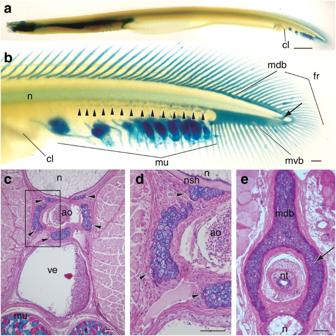Figure 1: The putative vertebral elements ofE. burgeri. (a) Lateral views of whole-mount Alcian blue-stained adult hagfish. Anterior is to the left. (b) This high-magnification view of the caudal fin area shows small cartilaginous nodules (the putative vertebral elements) located on the ventral side of the notochord at the post-cloacal level (arrowheads). More posteriorly, dorsal and ventral fin rays are connected with median cartilaginous plates, previously called 'median dorsal and ventral bars'18. (c–e) Transverse views of paraffin sections ofE. burgeristained with haematoxylin and eosin and Alcian blue. (c) The putative vertebral elements (arrowheads) are located ventral to the notochord surrounding the dorsal aorta at the post-cloacal region. (d) Higher magnification of the box shown inc. (e) The median dorsal bar is attached to a pair of cartilaginous arches on both sides of the notochord at the caudalmost level (arrow). ao, dorsal aorta; cl, cloaca; fr, fin ray; mdb, median dorsal bar; mu, mucus gland; mvb, median ventral bar; n, notochord; nsh, notochordal sheath; nt, neural tube; ve, vein. Scale bars, 1 cm (a); 1 mm (b); 100 μm (c–e). Figure 1: The putative vertebral elements of E. burgeri . ( a ) Lateral views of whole-mount Alcian blue-stained adult hagfish. Anterior is to the left. ( b ) This high-magnification view of the caudal fin area shows small cartilaginous nodules (the putative vertebral elements) located on the ventral side of the notochord at the post-cloacal level (arrowheads). More posteriorly, dorsal and ventral fin rays are connected with median cartilaginous plates, previously called 'median dorsal and ventral bars' [18] . ( c – e ) Transverse views of paraffin sections of E. burgeri stained with haematoxylin and eosin and Alcian blue. ( c ) The putative vertebral elements (arrowheads) are located ventral to the notochord surrounding the dorsal aorta at the post-cloacal region. ( d ) Higher magnification of the box shown in c . ( e ) The median dorsal bar is attached to a pair of cartilaginous arches on both sides of the notochord at the caudalmost level (arrow). ao, dorsal aorta; cl, cloaca; fr, fin ray; mdb, median dorsal bar; mu, mucus gland; mvb, median ventral bar; n, notochord; nsh, notochordal sheath; nt, neural tube; ve, vein. Scale bars, 1 cm ( a ); 1 mm ( b ); 100 μm ( c – e ). 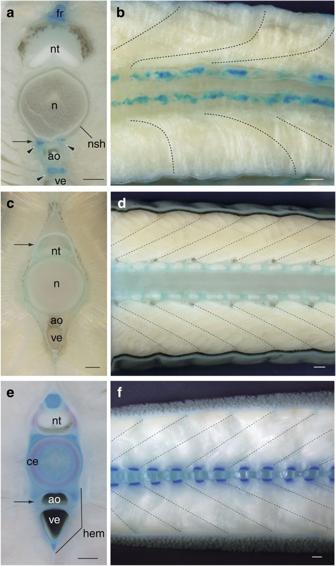Figure 2: Comparison of axial skeletal elements. (a–f) Transverse and horizontal sections of a whole-mount hagfish (E. burgeri), a lamprey (Lethenteron japonicum) and a catshark (Galeus nipponesis). (a) A transverse view ofE. burgeri. (b) Ventral view of a horizontally sectionedE. burgerispecimen. (c) Transverse view ofL. japonicum. (d) Ventral view of a horizontally sectionedL. japonicumspecimen. (e) Transverse view ofG. nipponesis. (f) Ventral view of a horizontally sectionedG. nipponesisspecimen. The levels of the horizontal sections in each specimen are indicated by arrows ina,c, ande. The ventral view of the horizontally sectionedE. burgeri(b) shows an asymmetric and non-metameric distribution of cartilaginous nodules along the anterior–posterior axis. Myosepta are indicated by broken lines. The dorsal view of the sectioned lamprey (d) shows dorsal vertebral elements segmentally arranged in register with myomeres. The ventral view of the horizontal section of the shark (f) shows a clear metameric distribution of the hemal arches. These horizontal sections of the lamprey and the shark show that two cartilaginous nodules are located between two myosepta along the anterior–posterior axis (d,f). ao, dorsal aorta; ce, centrum; fr, fin ray; hem, hemal arch; n, notochord; nsh, notochordal sheath; nt, neural tube; ve, vein. Scale bars, 1 mm. Full size image Figure 2: Comparison of axial skeletal elements. ( a – f ) Transverse and horizontal sections of a whole-mount hagfish ( E. burgeri ), a lamprey ( Lethenteron japonicum ) and a catshark ( Galeus nipponesis ). ( a ) A transverse view of E. burgeri . ( b ) Ventral view of a horizontally sectioned E. burgeri specimen. ( c ) Transverse view of L. japonicum . ( d ) Ventral view of a horizontally sectioned L. japonicum specimen. ( e ) Transverse view of G. nipponesis . ( f ) Ventral view of a horizontally sectioned G. nipponesis specimen. The levels of the horizontal sections in each specimen are indicated by arrows in a , c , and e . The ventral view of the horizontally sectioned E. burgeri ( b ) shows an asymmetric and non-metameric distribution of cartilaginous nodules along the anterior–posterior axis. Myosepta are indicated by broken lines. The dorsal view of the sectioned lamprey ( d ) shows dorsal vertebral elements segmentally arranged in register with myomeres. The ventral view of the horizontal section of the shark ( f ) shows a clear metameric distribution of the hemal arches. These horizontal sections of the lamprey and the shark show that two cartilaginous nodules are located between two myosepta along the anterior–posterior axis ( d , f ). ao, dorsal aorta; ce, centrum; fr, fin ray; hem, hemal arch; n, notochord; nsh, notochordal sheath; nt, neural tube; ve, vein. Scale bars, 1 mm. Full size image Somites and their derivatives To examine possible developmental similarities in putative vertebral elements between the hagfish and gnathostome vertebrae, we observed their embryonic development. Although we previously succeeded in collecting several early-stage hagfish embryos [20] , these were insufficient to trace the developmental processes of the somites and their derivatives. Hence, we conducted long-term incubation of fertilized hagfish eggs (Methods), and obtained 42 fertilized eggs at various developmental stages ( Supplementary Table S1 ). We selected three different stages of hagfish embryo, designated the early-, middle-, and late-pharyngula stages, for analysis of somite development ( Fig. 3 ; Supplementary Table S1 ). We used these three embryos to conduct detailed histological observations and used in situ hybridization to detect expression of Twist and Pax1/9 homologues ( Figs 3 and 4a–l ; Supplementary Figs S2 and S3 ), known to be specifically expressed in the sclerotomes of some gnathostomes [12] . 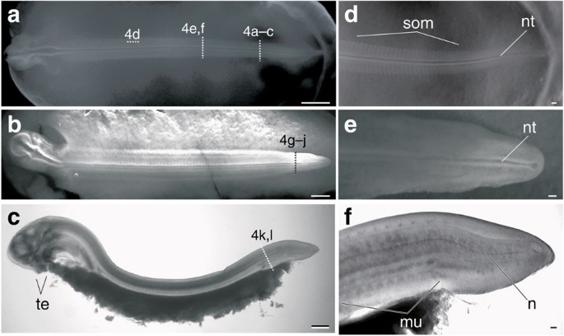Figure 3: Three stages ofE. burgeriembryos. (a–c) Whole-mount cleared embryos ofE. burgeri: (a) dorsal view of a 121 dpd embryo (early pharyngula); (b) dorsal view of a 145 dpd embryo (middle pharyngula); (c) lateral view of a 150 dpd embryo (late pharyngula) with tentacles and laterally flattened tail. (d–f) High-magnification view of the caudal regions: (d) early pharyngula embryo showing an epithelial somite; (e) middle pharyngula embryo; (f) late pharyngula embryo. Dotted lines indicate the levels of sections shown inFigure 3a–j. mu, mucus gland; nt, neural tube; som, somite; tent, tentacles. Scale bars, 1 mm (a–c); 100 μm (d–f). Figure 3: Three stages of E. burgeri embryos. ( a – c ) Whole-mount cleared embryos of E. burgeri : ( a ) dorsal view of a 121 dpd embryo (early pharyngula); ( b ) dorsal view of a 145 dpd embryo (middle pharyngula); ( c ) lateral view of a 150 dpd embryo (late pharyngula) with tentacles and laterally flattened tail. ( d – f ) High-magnification view of the caudal regions: ( d ) early pharyngula embryo showing an epithelial somite; ( e ) middle pharyngula embryo; ( f ) late pharyngula embryo. Dotted lines indicate the levels of sections shown in Figure 3a–j . mu, mucus gland; nt, neural tube; som, somite; tent, tentacles. Scale bars, 1 mm ( a – c ); 100 μm ( d – f ). 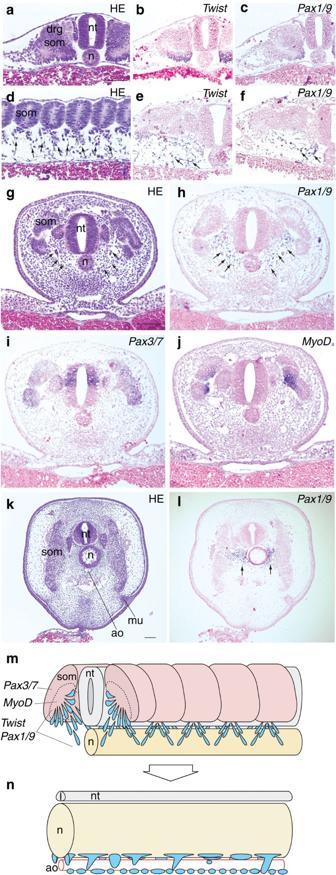Figure 4: Somite derivatives ofE. burgeri. (a–f) Early pharyngula. (a) Epithelial somite in the caudalmost region of the trunk. (b)Twistis strongly expressed in the ventral somite. (c)Pax1/9is weakly expressed in the median ventral somite. (d) Sagittal section showing rostrocaudally migrating putative sclerotomal cells at the anterior level of the trunk. (e,f) Transverse sections at the anterior level of the trunk showing migrating putative sclerotomal cells expressingTwist(e) andPax1/9(f) (arrowheads). (g–j) Middle pharyngula. (g) Mesenchymal cells located at the lateral side of the notochord. (h)Pax1/9expression by mesenchymal cells. (i)Pax3/7expression on the lateral side of a somite. (j)MyoDis strongly expressed at the medial side of a somite. (k,l) Late pharyngula. (k) Mesenchymal cells located at the dorsal aorta and the lateral side of the notochord. (l) Clear expression ofPax1/9is evident in the late pharyngula. (m,n) Schematic summary of the development of putative vertebral elements. (m) Medial ventral somites differentiate into mesenchymal cells (blue) in the early pharyngula. (n) The mesenchymal cells differentiate into the cartilaginous nodules in the adult. ao, dorsal aorta; mu, mucus gland; n, notochord; nt, neural tube; sc, sclerotome; som, somite. Arrows indicate the migrating sclerotomes. Scale bars, 100 μm. Full size image Figure 4: Somite derivatives of E. burgeri . ( a – f ) Early pharyngula. ( a ) Epithelial somite in the caudalmost region of the trunk. ( b ) Twist is strongly expressed in the ventral somite. ( c ) Pax1/9 is weakly expressed in the median ventral somite. ( d ) Sagittal section showing rostrocaudally migrating putative sclerotomal cells at the anterior level of the trunk. ( e , f ) Transverse sections at the anterior level of the trunk showing migrating putative sclerotomal cells expressing Twist ( e ) and Pax1/9 ( f ) (arrowheads). ( g – j ) Middle pharyngula. ( g ) Mesenchymal cells located at the lateral side of the notochord. ( h ) Pax1/9 expression by mesenchymal cells. ( i ) Pax3/7 expression on the lateral side of a somite. ( j ) MyoD is strongly expressed at the medial side of a somite. ( k , l ) Late pharyngula. ( k ) Mesenchymal cells located at the dorsal aorta and the lateral side of the notochord. ( l ) Clear expression of Pax1/9 is evident in the late pharyngula. ( m , n ) Schematic summary of the development of putative vertebral elements. ( m ) Medial ventral somites differentiate into mesenchymal cells (blue) in the early pharyngula. ( n ) The mesenchymal cells differentiate into the cartilaginous nodules in the adult. ao, dorsal aorta; mu, mucus gland; n, notochord; nt, neural tube; sc, sclerotome; som, somite. Arrows indicate the migrating sclerotomes. Scale bars, 100 μm. Full size image The early pharyngula of the hagfish developed less than 80 somites, which showed several different phases that enabled us to investigate the somitic differentiation process along the anterior–posterior embryonic axis ( Figs 3a,d and 4a–f ). At the level of the 60th to 70th somites, the ventromedial region of the epithelial somite, located at the lateral aspect of the notochord, expressed Twist and Pax1/9 genes ( Fig. 4b,c ), and at the level of the 30th to 40th somites, mesenchymal cells expressed the same genes at the ventromedial side around the notochord ( Fig. 4d–f ). We also observed that these mesenchymal cells (ventromedial cells) are subdivided into rostral and caudal populations, showing metameric patterning ( Fig. 4d ), as in some gnathostome sclerotomes [4] . However, this segmental pattern did not appear to be maintained in the adult cartilaginous state, as noted above ( Fig. 2a,b ). Most of the trunk somites had formed by the middle pharyngula stage ( Fig. 3b ). We thus observed caudal somite derivatives (80th somite level) in the prospective post-cloacal region wherein the putative vertebrae differentiate ( Fig. 3e ). Histological observations at the caudal levels in this stage showed epithelial somites and mesenchymal cells at the lateral aspect of the neural tube and notochord ( Fig. 4g ). Expression of Pax1/9 and Twist were also observed in those cells at caudal levels in the middle pharyngula stage ( Fig. 4h ). In particular, Twist expression was observed extensively in mesenchyme ventral to the notochord ( Supplementary Fig. S4 ), whereas Pax1/9 expression was restricted to the abovementioned ventromedial cells at the caudal level in this stage ( Fig. 4h ). The dorsolateral epithelial portion of the somites consistently expressed Pax3/7 and MyoD , which are expressed in the dermomyotome and myotome, respectively, in gnathostomes ( Fig. 4i,j ; Supplementary Fig. S5 ) [21] , [22] . These two genes showed mutually exclusive expression in these mesodermal cells. Similar to their gnathostome cognates [21] , [22] , Pax3/7 expression was detected in the lateral part of the somites, whereas MyoD expression was restricted to the medioventral region ( Fig. 4i,j ). This shows that dermomyotome and myotomal primodia can be identified as derivatives of a hagfish somite, with corresponding gene expression patterns and in comparable mediolateral relative positions to those in gnathostomes ( Fig. 4i,j ) [21] , [22] . Furthermore, these are found at the same axial level as that from which the putative vertebral elements are formed ( Fig. 1b ). This strongly suggests that the Pax1/9 -positive mesenchymal cells at the ventromedial aspect of the somite epithelia were developmentally equivalent to the sclerotome in gnathostomes ( Fig. 4h ) [12] , [21] , [22] . At the 90th somite level in the late pharyngula (the level of the vertebra-like elements; see Fig. 3c,f ), Pax1/9 -positive cells were distributed in more extensive domains than those in the previous embryo, with clusters detectable at the ventrolateral aspect of the notochord ( Fig. 3k,l ). This led us to infer that these Pax1/9 -positive cells may migrate further ventrally, surrounding the dorsal aorta, to differentiate into cartilaginous tissues on the ventral aspect of the notochord in later embryos ( Fig. 4m,n ). Given the metameric distribution patterns of the mesenchymal cells at the early pharyngula stage ( Fig. 4d ), the segmentally arranged sclerotomes, which originate from the ventromedial part of the somite ( Fig. 4a–c,e,f ), are likely to form the putative vertebral elements found in the adult ( Fig. 1 ) via molecular mechanisms common to those in gnathostomes ( Fig. 4m,n ) [12] , [21] , [22] . These results suggest that despite the minute size and disrupted segmental pattern of the putative vertebral elements in hagfish ( Fig. 1b–e ), they can be homologous to vertebrae. From the above observations, it seems plausible to assume that all the hagfish somites form sclerotomes and dermomyotomes at all axial levels in positions corresponding to those in gnathostomes, and that these somatic components arise via molecular developmental mechanisms similar to those in gnathostome embryos ( Fig. 4 ). At the post-cloacal level, the sclerotome-derived cells are distributed in regions prospectively occupied by the vestigial cartilaginous nodules in adults. Thus, in the hagfish, the somite appears to respond to signals derived from the notochord to specify cells destined towards skeletal differentiation. In this connection, the potential skeletogenic property of hagfish paraxial mesoderm is suggested in the chordal cranium (the caudal portion of the neurocranium known as the parachordals; Supplementary Fig. S6 ) [23] , [24] . Therefore, it seems likely that the notochordally derived signal is primarily capable of inducing chondrification in the paraxial mesoderm of the hagfish, and that this mechanism is lost secondarily from the pre-cloacal part of the hagfish trunk. Our observations are consistent at the anatomical and developmental level with the presence of axial cartilage in hagfish that is homologous to gnathostome vertebrae. This indicates that the presence of cartilaginous axial skeletal elements can be considered as a characteristic common to gnathostomes, lampreys and hagfishes. Hence, we can no longer exclude the hagfish from the Vertebrata simply due to the absence of a cartilaginous axial skeleton, which has now been disproved ( Fig. 5 ). 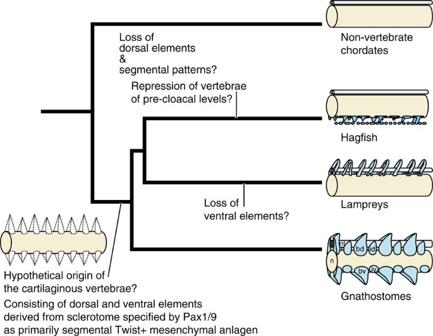Figure 5: Hypothetical scenario of vertebral evolution. This phylogenetic tree is based mainly on molecular data and hagfishes are clustered with lampreys as members of monophyletic cyclostomes25,26,27,28. The origins of the cartilaginous vertebrae, consisting of dorsal and ventral elements, as well as associated developmental mechanisms are assumed to have been obtained before the divergence of gnathostomes, lampreys, and hagfish. The vertebral elements of the extant vertebrates are coloured blue, and those of the common ancestor of entire extant vertebrates are indicated by dotted lines. bd, basi-dorsal; bv, basi-ventral; id, inter-dorsal; iv, inter-dorsal; n, notochord; nt, neural tube. Figure 5: Hypothetical scenario of vertebral evolution. This phylogenetic tree is based mainly on molecular data and hagfishes are clustered with lampreys as members of monophyletic cyclostomes [25] , [26] , [27] , [28] . The origins of the cartilaginous vertebrae, consisting of dorsal and ventral elements, as well as associated developmental mechanisms are assumed to have been obtained before the divergence of gnathostomes, lampreys, and hagfish. The vertebral elements of the extant vertebrates are coloured blue, and those of the common ancestor of entire extant vertebrates are indicated by dotted lines. bd, basi-dorsal; bv, basi-ventral; id, inter-dorsal; iv, inter-dorsal; n, notochord; nt, neural tube. Full size image Although our developmental study suggested a sclerotomal origin for the ventral elements, the origin of the dorsal element, reminiscent of the neural arches and spine of gnathostomes, remains unclear ( Fig. 1b ). Nevertheless, given the anatomical similarity of this element to the gnathostome counterpart ( Figs 1e and 2e,f ), it is highly possible that they share the same developmental patterns, suggesting that the paraxial mesoderm of the entire common ancestor of gnathostomes, lampreys and hagfishes could form cartilaginous elements on both the dorsal and ventral sides of the notochord. Taking into account the recently reconstructed phylogenetic trees based on molecular data, which support a monophyly of hagfishes and lampreys [25] , [26] , [27] , [28] , it seems reasonable to hypothesize that the dorsal and ventral vertebral elements were obtained from a common ancestor of the entire vertebrates, and that subsequent secondary losses would have led to loss of the dorsal vertebral elements in the hagfishes on one hand, and to a ventral vertebral element in the lamprey on the other ( Fig. 5 ). To test this hypothesis, further comparative developmental studies will be required to exclude the possibility of independent evolutionary occurrence of vertebral elements in the extant agnathan lineages, because it is still unclear whether the entire part of the vertebral elements of extant agnathans is derived from sclerotomal cells, as occurs in gnathostomes [12] . We still cannot rule out completely the possibility that some parts of the vertebral elements of lamprey and hagfish are derived from non-sclerotomal cells (for example, neural crest cells). Finally, it remains to be determined whether the morphological pattern of hagfish axial skeletal elements represents a secondary loss of segmentation or an ancestral state before acquisition of the segmental pattern. However, the former scenario is more plausible under the assumption of the monophyly of the extant agnathans ( Fig. 5 ). This scenario implies that the common ancestor of the extant gnathostomes and agnathans had the developmental mechanism to form a segmental axial skeleton consisting of two topographically different cartilaginous nodules, one located at the level of the myoseptum and the other at the intermediate level between the two myosepta, along the anterior–posterior axis, as seen in the vertebral elements of lampreys and gnathostomes ( Figs 2 and 5 ). The origin of this developmental mechanism could date back to around 500 million years ago based on the divergence time between agnathans and gnathostomes [26] , [27] . Also problematic is the absence of cartilaginous tissue from the pre-cloacal trunk, as well as the absence of dorsal skeletal elements in most of the post-cloacal region ( Fig. 1 ). Further study is required to elucidate whether such a loss can be simply explained by adaptation to a hagfish lifestyle or by the long evolutionary period [2] . The origin of the axial skeleton remains an issue in evolutionary developmental biology, and will require consideration of paleontological, embryological and molecular data [12] , [13] , [25] , [26] , [27] , [28] , [29] , [30] . We are hopeful that further advances in hagfish embryology will provide more insights into the evolution of the axial skeletal element in the early vertebrates, especially into the origin of its segmental pattern. Sample collection and aquarium maintenance Adult males and females of E. burgeri were collected using eel traps from a depth of 25–100 m in the Japan Sea off the Shimane and Yamaguchi prefectures during September and October. After the hagfish were transferred to a laboratory aquarium (at 16 °C) and sexed by manipulation, about 100 adult specimens were maintained in an aquarium tank lined with potentially favourable substrates, including fine-grain sand and oyster shells (1,000 l, 16–17 °C) (refs 31 , 32 ). The deposited eggs were individually incubated in a plastic container (4 cm×4 cm×5 cm) in the same aquarium tank [32] . Fertilized eggs were identified by visual inspection and were prepared for further analysis. All of the embryos are listed in Supplementary Table S1 . Molecular cloning Total RNA was extracted from embryos using TRIZOL reagent (Invitrogen). Degenerated RT–PCR was performed to amplify fragments of Twist , Pax1/9 , and MyoD messenger RNA using the primer sets listed in Supplementary Table S2 . These fragments were isolated using the TOPO TA Cloning Kit Dual Promoter (Invitrogen) and sequenced using an ABI 3130XL automated sequencer (Applied Biosystems). The sequence data were submitted to the DDBJ database (AB594746, AB594747, AB594748). To identify the orthologous genes of the isolated fragments, comparable sequence data were surveyed using the NCBI protein database and a BLAST search, and multiple sequence alignments were generated using the CLUSTALW multiple alignment program [33] . Multiple sequence alignments were corrected by visual inspection. Based on these alignments, gene-specific residues and motifs were identified ( Supplementary Figs S3 , S4 , S6 ). Histology and in situ hybridization Hagfish specimens were fixed in Serra's fixatives for 24–48 h, dehydrated using an ethanol series, placed in xylene, embedded in paraffin, and sliced at a thickness of 8 μm. The sliced sections were deparaffinized and stained with haematoxylin, eosin and Alcian blue [34] . In situ hybridization was carried out using a Ventana automated machine (Ventana Medical Systems). Detection of signals and counterstaining were performed using the BlueMap NBT/BCIP substrate kit and the nuclear fast red equivalent reagent, ISH RED (Ventana). Accession codes: The sequence data have been deposited to the DDBJ database under accession codes AB594746 , AB594747 and AB594748 . How to cite this article: Ota, K. G. et al . Identification of vertebra-like elements and their possible differentiation from sclerotomes in the hagfish. Nat. Commun. 2:373 doi: 10.1038/ncomms1355 (2011).